Lifetime blinking in nonblinking nanocrystal quantum dots Nanocrystal quantum dots are attractive materials for applications as nanoscale light sources. One impediment to these applications is fluctuations of single-dot emission intensity, known as blinking. Recent progress in colloidal synthesis has produced nonblinking nanocrystals; however, the physics underlying blinking suppression remains unclear. Here we find that ultra-thick-shell CdSe/CdS nanocrystals can exhibit pronounced fluctuations in the emission lifetimes (lifetime blinking), despite stable nonblinking emission intensity. We demonstrate that lifetime variations are due to switching between the neutral and negatively charged state of the nanocrystal. Negative charging results in faster radiative decay but does not appreciably change the overall emission intensity because of suppressed nonradiative Auger recombination for negative trions. The Auger process involving excitation of a hole (positive trion pathway) remains efficient and is responsible for charging with excess electrons, which occurs via Auger-assisted ionization of biexcitons accompanied by ejection of holes. Photoluminescence (PL) intermittency, or PL blinking, is a common property of nanoscale light emitters [1] . Nanocrystal quantum dots (NQDs) have often been used as model systems in studies of this intriguing phenomenon [2] . A majority of existing models relate PL intensity blinking to random charging/discharging of the NQD core [3] , [4] . However, several studies have pointed towards other possible mechanisms for intensity fluctuations [5] , [6] that can be linked, for example, to surface recombination centres [7] , [8] . Specifically, we have recently shown that, in addition to charging/discharging of the NQD core (A-type blinking), PL intensity fluctuations can be caused by random variations in occupancy of surface related hot-electron traps that, if unoccupied, intercept a photoexcited electron before its relaxation to the band-edge emitting state (B-type blinking) [8] . During A-type intensity blinking, when one or more additional charges are present in the NQD core, fast nonradiative Auger recombination quenches PL, which would correspond to a weakly emitting (dark) state as illustrated in Fig. 1a . In CdSe nanocrystals overcoated with ~7 to 11 monolayers of crystalline CdS, a higher emissivity grey state with a moderate PL quantum yield [9] of ~10% has been observed. This state was attributed to a charged exciton whose emission was enhanced relative to core-only nanocrystals owing to a reduced Auger decay rate [10] , [11] . For very thick shells (~15 to 19 monolayers), a complete suppression of blinking can be achieved for individual NQDs [12] . This might imply either a complete elimination of charge fluctuations within the NQD or the realization of a regime where charge fluctuations do not noticeably change the emission intensity. The latter is possible when Auger recombination is significantly suppressed and hence the emission quantum yield of charged excitons approaches that of the neutral excitons ( Fig. 1b ). Recently, several groups have reported nonblinking NQDs [13] , [14] , [15] , [16] ; however, it still remains unclear which of the above two regimes has been realized in these structures. 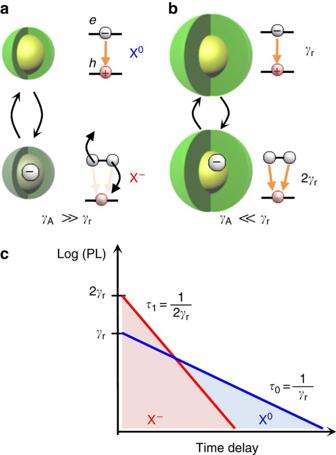Figure 1: Relationship between charging and blinking in thin-shell and thick-shell CdSe/CdS NQDs. (a) In thin-shell NQDs, the high-emissivity 'bright' state corresponds to an exciton in a neutral dot (X0). The dominant recombination channel is radiative decay (orange arrow) with rateγr. Any random fluctuation towards a charged state (here a negative trion X−) renders the dot essentially non-emissive (the dot blinks off) because the rate of nonradiative Auger recombination (black arrows; rateγA) is orders of magnitude higher thanγr. (b) The core/shell NQDs with very thick shells (≥15 monolayers) are essentially nonblinking (the PL intensity remains stable over minutes and even hours). This behaviour can be either due to a complete suppression of charge fluctuations (the dot is always in the neutral state) or owing to the fact that the PL quantum yield of charged excitons is similar to that of neutral excitons. The latter situation can only be realized if the Auger recombination rate,γA, of a charged exciton is much lower than its radiative decay rate. (c) The expected qualitative form of the PL decay traces (semi-log scale) for the neutral and the charged exciton. Because the number of radiative recombination pathways is increased in the presence of an additional electron, the radiative lifetime of a trion is twice as short as that of a neutral exciton (radiative rate 2γr). Further, because of the increase in the emission rate, the early time PL amplitude of the trion is also increased by a factor of two compared with that of the neutral exciton. By analysing lifetime variations, one can, in principle, determine whether different charged states contribute to the measured emission even when the PL intensity is nonblinking. Figure 1: Relationship between charging and blinking in thin-shell and thick-shell CdSe/CdS NQDs. ( a ) In thin-shell NQDs, the high-emissivity 'bright' state corresponds to an exciton in a neutral dot ( X 0 ). The dominant recombination channel is radiative decay (orange arrow) with rate γ r . Any random fluctuation towards a charged state (here a negative trion X − ) renders the dot essentially non-emissive (the dot blinks off) because the rate of nonradiative Auger recombination (black arrows; rate γ A ) is orders of magnitude higher than γ r . ( b ) The core/shell NQDs with very thick shells (≥15 monolayers) are essentially nonblinking (the PL intensity remains stable over minutes and even hours). This behaviour can be either due to a complete suppression of charge fluctuations (the dot is always in the neutral state) or owing to the fact that the PL quantum yield of charged excitons is similar to that of neutral excitons. The latter situation can only be realized if the Auger recombination rate, γ A , of a charged exciton is much lower than its radiative decay rate. ( c ) The expected qualitative form of the PL decay traces (semi-log scale) for the neutral and the charged exciton. Because the number of radiative recombination pathways is increased in the presence of an additional electron, the radiative lifetime of a trion is twice as short as that of a neutral exciton (radiative rate 2γ r ). Further, because of the increase in the emission rate, the early time PL amplitude of the trion is also increased by a factor of two compared with that of the neutral exciton. By analysing lifetime variations, one can, in principle, determine whether different charged states contribute to the measured emission even when the PL intensity is nonblinking. Full size image Here we investigate a new type of nonblinking thick-shell CdSe/CdS nanocrystals (giant NQDs) [12] , [16] and discover a new regime of emission where discrete fluctuations in the PL lifetime (lifetime blinking) occur without appreciable changes in the PL intensity. This phenomenon, illustrated in Fig. 1b,c , is observed at least to some extent in all giant NQDs analysed in this study (~40 nanocrystals from 2 synthesized batches). Single-dot measurements under controlled electrochemical charge injection yield the PL lifetimes of neutral and charged excitons. On the basis of these data, we can unambiguously attribute the observed lifetime blinking to switching of the nanocrystal between the neutral and the negatively charged state. Although, in standard nanocrystals, charged excitons (trions) are virtually nonemissive because of fast nonradiative Auger decay, the Auger process is significantly suppressed in giant NQDs, especially for negative trions. As a result, charging of the nanocrystal with additional electrons does modify the radiative lifetime but not the emission intensity. Auger decay suppression is less efficient for positive trions; therefore, when photoexcitation produces a biexciton, its recombination is dominated by the Auger decay channel in which the electron-hole pair recombination energy is transferred to a hole. Occasionally, the hole is ejected via this positive-trion Auger recombination pathway, which leads to ionization of the NQD. We find that this process is primarily responsible for NQD charging with excess electrons. Experimental set-up In our studies, we use a custom-built electrochemical cell incorporated into a micro-PL system based on a confocal microscope (see Methods) [8] , [17] . On the basis of the normalized amplitude of the zero-delay ( t =0) feature in the intensity auto-correlation function g (2) ( Fig. 2a inset), we verified that the detected signal originated from a single NQD ( g (2) (0)<0.5 implies a single quantum emitter) [18] . PL time trajectories were acquired under pulsed excitation in a time-tagged, time-resolved mode. The delay between each detection event and the excitation pulse (micro-time) was recorded with an overall resolution of 300 ps. In addition, we also monitored the time elapsed since the start of the experiment (macro-time). After choosing an appropriate bin size (100–200 ms in our measurements), a PL decay histogram and a mean PL intensity were calculated for each bin time. To evaluate the average PL lifetime for a given bin, we calculated the weighted average of the micro-times histogram. This allowed for a fast and reliable estimation of the PL lifetime without any fitting or a priori assumption on the PL dynamics (for example, single- versus multi-exponential). 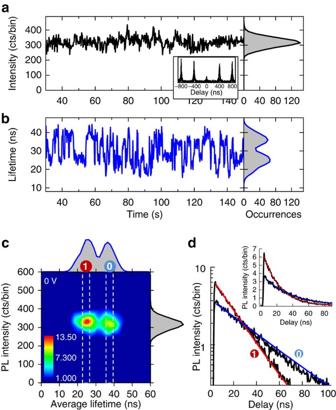Figure 2: Discrete charge fluctuations in a single nonblinking NQD. Time-tagged, time-resolved data from an individual NQD acquired at low fluence (the average NQD occupancyNex~0.08) under zero electrochemical potential (0 V vs silver wire reference) and analysed with a time bin of 200 ms. (a) PL intensity and (b) average lifetime trajectories. The histograms obtained for the total experiment time of 180 s are also shown. Inset: autocorrelation function measured in a Hanbury Brown and Twiss configuration. The area of the central peak divided by the mean area of the side peaks yieldsg(2)(0)=0.1±0.01. (c) The corresponding FLID colour plot. The two-dimensional histogram was constructed with a 1-ns lifetime binning and a 15 counts intensity binning, smoothened by a two-point averaging. The colour scale represents the frequency of occurrences of given intensity-lifetime pairs. (d) The PL decay curves obtained by filtering the bins in windows (0) and (1) marked in (b) normalized to the total number of the selected bins. The blue and red curves show the mono-exponential fits with lifetimes 39 ns (0) and 19 ns (1), respectively. The inset is the same plot but on a linear scale to show more clearly the factor of ~2 difference between the early time PL amplitudes, as expected for the neutral and singly-charged exciton states. Figure 2: Discrete charge fluctuations in a single nonblinking NQD. Time-tagged, time-resolved data from an individual NQD acquired at low fluence (the average NQD occupancy N ex ~0.08) under zero electrochemical potential (0 V vs silver wire reference) and analysed with a time bin of 200 ms. ( a ) PL intensity and ( b ) average lifetime trajectories. The histograms obtained for the total experiment time of 180 s are also shown. Inset: autocorrelation function measured in a Hanbury Brown and Twiss configuration. The area of the central peak divided by the mean area of the side peaks yields g (2) (0)=0.1±0.01. ( c ) The corresponding FLID colour plot. The two-dimensional histogram was constructed with a 1-ns lifetime binning and a 15 counts intensity binning, smoothened by a two-point averaging. The colour scale represents the frequency of occurrences of given intensity-lifetime pairs. ( d ) The PL decay curves obtained by filtering the bins in windows (0) and (1) marked in ( b ) normalized to the total number of the selected bins. The blue and red curves show the mono-exponential fits with lifetimes 39 ns (0) and 19 ns (1), respectively. The inset is the same plot but on a linear scale to show more clearly the factor of ~2 difference between the early time PL amplitudes, as expected for the neutral and singly-charged exciton states. Full size image Lifetime blinking In Fig. 2a,b , we show the PL intensity and lifetime trajectories from an individual CdSe/CdS giant NQD (15 monolayer thick shell) obtained with a bin size of 200 ms. The PL intensity (upper black trace) is stable over the entire experiment (180 s) and is characterized by a nearly Poissonian, single-peak distribution ( Supplementary Fig. S1 ). This is a typical example of nonblinking behaviour, suggestive of emission from a single, well-defined state. The inspection of a lifetime trajectory, however, indicates the involvement of at least two different states with two distinct lifetimes. Indeed, the lifetime trajectory ( Fig. 2b ) exhibits jumps between two values, leading to a double-peak distribution. Figure 2c shows the same set of data using the fluorescence lifetime–intensity distribution (FLID) representation. The colour scale is used to show the frequency of occurrence of bins with a given pair of intensity ( y axis) and lifetime ( x axis). The FLID clearly indicates that two different states contribute to the PL, with almost equal weight for this particular NQD. Further evidence for the two-state character of emission comes from the analysis of lifetime-filtered decay curves that are constructed by selecting all bins whose average lifetime falls within either window (1) or (0) in the FLID in Fig. 2c (dashed lines). The histograms of the micro-times from all selected bins are summed to form the PL decay curves shown in Fig. 2d . We fit the two decay curves of Fig. 2d to mono-exponential decays and obtain the two lifetimes τ 1 =19 ns and τ 0 =39 ns. These fitted lifetimes differ from the apparent values in Fig. 2c because the FLID is constructed using a weighted-average formula but not an exponential fitting. Because the PL quantum yields of states (1) and (0) are nearly identical, the shortening of the PL lifetime by a factor τ 0 / τ 1 ~2 must be accompanied by an equal increase in the radiative recombination rate. Indeed, we observe that the initial amplitude of trace (1) is nearly twice as large as the amplitude of trace (0) ( Fig. 2d , inset). Origin of lifetime fluctuations Recently, PL fluctuations were studied in the so-called dot-in-a-rod nanostructures, that have a similar composition (CdSe/CdS) but a different morphology [19] . They were attributed to switching in localization of the photoexcited electron between the core and the rod-shaped shell [19] , on the basis of the observed correlated changes in the PL intensity, wavelength and linewidth. In our giant NQDs, however, lifetime variations are not accompanied by measurable PL intensity or wavelength fluctuations, suggesting a different underlying mechanism. A possible explanation of the observed lifetime fluctuations is in terms of charging as illustrated in Fig. 1b,c . The addition of a charge (an electron in Fig. 1b ) to a neutral exciton state doubles the number of radiative recombination pathways, and therefore increases the radiative decay rate by a factor of two [20] . This can explain our observation of an approximately twofold decrease in the PL relaxation time. The radiative decay rate also determines the instantaneous PL intensity; therefore, the radiative lifetime-shortening should be accompanied by a proportional increase in the PL signal amplitude, which is again in accord with our experimental observations. As was mentioned earlier, an important condition for these observations is a significant suppression of nonradiative Auger recombination (see following subsection), which results in the regime where the recombination of charged species is dominated by the radiative process. To verify the hypothesis of charging being responsible for the lifetime fluctuations, we investigate the effect of controlled electrochemical charge injection [8] , [17] , [21] on PL intensities and relaxation rates. In Fig. 3a-c , we show FLIDs that are obtained for 3 values of applied potential 0, −0.5, and −0.8 V (panels a, b, c, respectively). This corresponds to a progressively higher position of the Fermi level, favouring the injection of electrons into the nanocrystal. At 0 V (panel a), we observe the two-lobe distribution described in the previous paragraph. At −0.5 V (panel b), the PL lifetime distribution shifts towards state (1) with the faster PL decay τ 1 , suggesting that this state is a negatively charged exciton (negative trion). As discussed above, on the basis of the number of available radiative recombination pathways [20] , [22] (see Methods and Fig. 1c ), the radiative lifetime of the negative trion is expected to be twice as short as that of the neutral exciton, which is indeed in close agreement with our data. This further indicates that, in the case of a negative trion, the Auger process is slow compared with radiative recombination. Therefore, introduction of an additional electron during NQD charging does not lead to the reduction of the PL quantum yield, which explains the observed behaviour—the drop in the lifetime occurs without changes in the PL intensity. This observation is consistent with a significant suppression of Auger decay in giant NQDs observed in refs 10 , 11 and is confirmed by the statistical analysis of a large number of giant NQDs shown in Supplementary Fig. S2 . Under a more negative potential of −0.8 V ( Fig. 3c ; Supplementary Fig. S3 ), we observe a further shortening of the lifetime, again without any noticeable change in the PL quantum yield. This can be attributed to the formation of a doubly charged exciton. 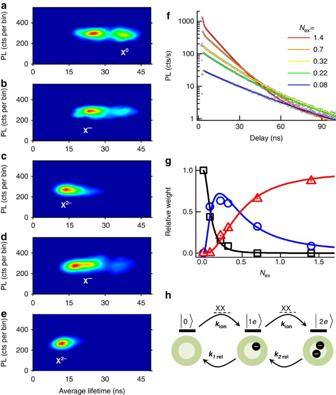Figure 3: Electrochemical and photoinduced charging of a single NQD. Data are from the same NQD used earlier. (a–c) FLIDs under increasing negative potential (electron injection) and constant fluence (Nex~0.08): (a) 0 V; (b)−0.5 V; and (c)−0.8 V. Bin size is 200 ms. (d,e) The potential is kept at zero but the fluence is increased: (d)Nex~0.22 (bin size 80 ms); (e)Nex~0.7 (bin size 30 ms). (f) PL decay curves acquired over 180 s under increasing fluence (open circles) and fits using a global fitting procedure described in the text (solid lines). (g) Open symbols: relative weights of emission from the neutral exciton (black squares), singly (blue circles) and doubly (red triangles) charged excitons extracted from the global fit parameters. Solid lines: simulated average populations for a neutral (black), singly (blue) and doubly (red) charged NQD states obtained using the model. (h) Schematics of the model for photoinduced charging. XX represents the creation of a biexciton on laser excitation, which can lead to Auger photoionization and charging of the nanocrystal with ratekion. A singly charged dot (state 1e) and a doubly charged dot (state 2e) relax by losing an electron with ratesk1 relandk2 rel, respectively. Figure 3: Electrochemical and photoinduced charging of a single NQD. Data are from the same NQD used earlier. ( a – c ) FLIDs under increasing negative potential (electron injection) and constant fluence ( N ex ~0.08): ( a ) 0 V; ( b ) − 0.5 V; and ( c ) − 0.8 V. Bin size is 200 ms. ( d , e ) The potential is kept at zero but the fluence is increased: ( d ) N ex ~0.22 (bin size 80 ms); ( e ) N ex ~0.7 (bin size 30 ms). ( f ) PL decay curves acquired over 180 s under increasing fluence (open circles) and fits using a global fitting procedure described in the text (solid lines). ( g ) Open symbols: relative weights of emission from the neutral exciton (black squares), singly (blue circles) and doubly (red triangles) charged excitons extracted from the global fit parameters. Solid lines: simulated average populations for a neutral (black), singly (blue) and doubly (red) charged NQD states obtained using the model. ( h ) Schematics of the model for photoinduced charging. XX represents the creation of a biexciton on laser excitation, which can lead to Auger photoionization and charging of the nanocrystal with rate k ion . A singly charged dot (state 1 e ) and a doubly charged dot (state 2 e ) relax by losing an electron with rates k 1 rel and k 2 rel , respectively. Full size image Auger recombination rates of negative and positive trions Interestingly, despite a significant suppression of Auger recombination for negative trions, the Auger recombination of biexcitons in this giant NQD is still fast. The two-photon correlation measurements show that g (2) (0)/g (2) (T) ~0.1 ( T =400 ns is pulse-to-pulse separation) in the limit of low fluences ( Fig. 2a , inset). This indicates that the ratio of the biexciton to single-exciton quantum yield is ~0.1 (refs 24 , 25 ) and further implies a fairly fast Auger recombination with a time constant of ~1 ns. Indeed, the PL dynamics measured at a high fluence indicate a biexciton lifetime of ~0.8 ns (see Supplementary Fig. S4 ), which is about 10 times faster than the estimated biexciton radiative lifetime (see Methods). These observations suggest that, although Auger decay of the negative trion is suppressed in the giant NQDs, the Auger process in which the hole is excited (positive trion channel) is still efficient and it dominates biexciton recombination. The reasons for a considerable difference in the Auger decay rates of negative and positive trions might relate to a much higher density of hole states in II–VI NQDs [25] and/or a higher degree of spatial confinement for holes than for electrons in giant NQDs [11] , [26] . Because of the relatively small conduction-band offset at the CdSe/CdS interface (~100 meV) [26] , the electrons in giant NQDs are delocalized over the entire nanocrystal while holes are tightly confined to the CdSe core. Because Auger recombination rates scale as the inverse of the effective volume occupied by the carriers [27] , [28] , Auger decay involving excitation of a delocalized electron should be slower than the process involving a more tightly confined hole. A pronounced difference between the Auger decay rates of negative and positive trions may explain previous observations of significant dot-to-dot variations in the biexciton PL quantum yields among nominally identical nonblinking giant NQDs [24] . Even when Auger decay for the negative trion is suppressed, variations in the rate of the positive trion pathway may lead to a significant spread in the biexciton Auger time constants. Such variations can result from differences in the steepness of the core/shell confinement potential [11] , [29] as well as dot-to-dot variations in the core size. These are expected to affect more strongly a recombination channel involving excitation of the core-localized hole, compared with that with the excitation of the more delocalized electron. Charging mechanism Our measurements also help clarify the mechanism for charge fluctuations in these nanocrystals, which we believe is associated with Auger-assisted ionization, as suggested by Efros and Rosen [4] . Recently, Nesbitt and co-workers pointed out that even at very low excitation fluences, the Poissonian statistics of the excitation process lead to a significant probability for creating a multiexciton over typical experimental times [3] . The Auger decay of such a multiexciton can lead to the ejection of a charge, a phenomenon known as Auger ionization [30] . As we reasoned above, the more probable Auger decay pathway in these nanocrystals involves the excitation of a hole. As a result, Auger ionization is expected to produce primarily negatively charged nanocrystals. Further, as the probability of Auger ionization increases with increasing pump intensity so do the odds of detecting emission from the singly and doubly charged states. Indeed, when the laser fluence is increased at a fixed electrochemical potential ( Fig. 3a,d,e ), we observe a shift of the PL lifetime distribution towards the singly and then doubly charged negative excitons. This behaviour mimics the lifetime changes observed under electrochemical charging at a negative potential ( Fig. 3a–c ). Taken together, the results of spectro-electrochemical measurements and the pump-intensity-dependent studies suggest that lifetime blinking observed in these thick-shell NQDs is due to fluctuations between the neutral exciton state and the negative trion. To quantify the degree of photocharging, we perform a global fit of the PL decay curves measured for different pump fluences ( Fig. 3f ). We use a four-exponential function, in which the four shared time constants describe the decay of the neutral exciton, singly and doubly charged excitons and the biexciton. From these fits, the contribution of a particular state to PL over the duration of the experiment is obtained from the product Aτ, where τ is the PL lifetime of a given state and A is the corresponding amplitude. As neutral and negatively charged excitons have similar PL quantum yields, the values of Aτ provide a direct measure of the time spent by the nanocrystal in a given charge state. The results of this analysis are shown in Fig. 3g with open symbols. For increasing fluence, the nanocrystal spends an increasing amount of time first in the singly charged (up to N ex ~0.4; N ex is the average NQD exciton occupancy) and then in the doubly charged state. To model these observations, we assume that the photo-ionization rate k ion scales proportionally to the probability of creating a multiexciton of any order and can be calculated from k ion = a ion × , where P(n,N ex ) is the Poisson probability of exciting an n -exciton, if the average number of excitons generated per NQD is N ex . When the nanocrystal is promoted to a charged state, it can relax with rates k 1 rel and k 2 rel for singly and doubly charged excitons, respectively ( Fig. 3h ). We solve the steady-state rate equations to compute the time-averaged population in each state as a function of N ex . The simulated curves, shown by the solid lines in Fig. 3g , are in excellent agreement with the experimental data. The values of the two free parameters a 1,2 = a ion / k 1,2 rel used in this simulation are a 1 =250 and a 2 =14, implying that the relaxation rate of the doubly charged nanocrystal is ~18 times faster than for the singly charged nanocrystal. This suggests that a doubly charged state is less stable than a singly charged state, as expected under zero applied potential. In analogy with the analysis of the ON/OFF time statistics performed for traditional intensity blinking, we conduct a similar analysis for lifetime blinking by setting a lifetime threshold to distinguish between two different charge states (0) and (1). The results of this analysis for the data in Fig. 2b are shown in Supplementary Fig. S5 . They indicate that the distribution of times spent by the dot in a given charge state deviates from the power-law distribution typically observed for intensity blinking in standard NQDs [31] . The initial exponential drop in the probability with increasing event duration indicates that both charging and discharging rates are on the order of 1 s −1 at N ex ~ 0.1. This corresponds to an ionization probability a ion of ~10 −4 per multiexciton generation event, which is similar to the probability inferred in the studies of ref. 3 from the analysis of the ON-time distribution in blinking dots. A very small value of a ion suggests that Auger recombination in these nanocrystals only rarely results in ionization events. However, because of the slow rate of the NQD re-neutralization, such events can still be clearly observed in the measured lifetime trajectories. The presence of longer events exceeding a few seconds suggests that an additional ionization mechanism is probably contributing to the charge fluctuations. Long-lasting charging under high-energy blue or ultraviolet excitation was reported previously for CdSe nanocrystals [32] and has been recently studied in great detail for PbSe and PbS NQDs [33] . These earlier studies indicate the existence of long-lived surface/ligand-related traps that can efficiently intercept a hot carrier before its relaxation to the band-edge state. The charging resulting from this effect is characterized by relaxation times of up to tens of seconds [33] . To summarize, we observe that stable, nonblinking PL from thick-shell CdSe/CdS giant NQDs can be accompanied by significant fluctuations in PL lifetimes (lifetime blinking). On the basis of direct measurements of PL dynamics under controlled electrochemical charge injection, we conclude that the PL lifetime fluctuations are associated with random charging of the NQD with excess electrons. We further observe that the emission quantum yields of singly and doubly negatively charged excitons are similar to those of neutral excitons. Therefore, while having a pronounced effect on the emission lifetime, NQD charging does not lead to appreciable changes in the PL intensity, resulting in the apparent nonblinking behaviour. Pump-intensity-dependent measurements suggest that the nanocrystal charging is a photo-induced process associated with Auger recombination of biexcitons (Auger ionization) that are occasionally created even at very low excitation fluences [3] . The PL quantum yields of biexcitons can be up to ten times lower than those of single excitons and negative trions, which can be explained by a highly efficient Auger decay pathway involving excitation of a hole ('positive-trion' pathway). The greater rate of Auger decay of the positive trion compared with the negative trion is likely due to a higher density of valence-band states and/or a higher degree of spatial confinement for holes compared with electrons. This asymmetry in the Auger decay rates helps to rationalize the fact that photocharging produces mostly negatively charged nanocrystals. It may also explain previous observations indicating a large variability in the biexciton PL quantum yields among individual nonblinking giant NQDs from the same ensemble sample [24] . Even if Auger decay for the negative trion is suppressed in all NQDs, the rate of the positive trion pathway can be strongly dependent on small variations in the core size and/or in the degree of alloying at the core/shell interface [11] , owing to the tight confinement of the hole inside the NQD core. In contrast, the electron wavefunction is delocalized over the entire NQD volume, which makes the negative trion Auger rate almost insensitive to such variations and results in robust nonblinking behavior. Nanocrystal synthesis The synthesis of giant core/shell CdSe/CdS nanocrystals was performed using a modified version of the successive ionic layer adsorption and reaction method reported in ref. 34 . The original surface ligands were exchanged for mercaptoundecanoic acid using a procedure described in ref. 8 . Then, the NQDs were re-dissolved in distilled water and directly deposited from a very dilute solution onto an indium-tin-oxide-coated transparent working electrode. We used a platinum gauze attached to a platinum wire as a counter electrode. All potentials reported in this work are referenced to a silver wire quasi-reference. The experiments were performed using several combinations of solvents (acetonitrile or propylene carbonate) and supporting electrolytes (tetrabutylammonium perchlorate or lithium perchlorate; 0.1 M concentrations). We did not notice any dependence of the results on the identities of either the solvent or the supporting electrolyte. Photoluminescence measurements PL was excited by 60 ps, 405 nm laser pulses at 2.5 MHz repetition rate through an oil-immersion objective with a numerical aperture of 1.2. The average number of excitons generated per pulse per NQD, N ex , was estimated following ref. 24 . The collected PL was spectrally filtered and detected by a pair of fast avalanche photodiodes with 300 ps time resolution. We used a Hanbury Brown and Twiss configuration to measure the intensity auto-correlation function g (2) ( t ). Modelling of radiative and Auger decay rates We estimate the radiative and non-radiative decay rates of neutral and charged, single and bi-excitons using a statistical scaling approach, which considers the number of recombination pathways that lead from the initial to the final charge carrier configuration [21] , [23] . This approximation is expected to be valid for modelling room-temperature PL dynamics, when the bright-dark exciton splitting is small compared with the thermal energy k B T and spin selection rules do not have a major role. The radiative decay of the neutral exciton is denoted γ r , and we assume for simplicity that its PL quantum yield is unity, so that the PL lifetime is: We denote the Auger recombination rates of the negative (positive) trion as γ A − ( γ A + ). If we account for all possible carrier configurations and recombination pathways for the state i with n e electrons and n h holes, we obtain the following scaling for the radiative rate γ r i Applying this expression to the radiative rate of the negative trion, we obtain: The corresponding measured PL lifetime is: We use equations (1) and (4) to extract the Auger lifetime, 1/γ A − , from the PL lifetime measurements ( Supplementary Fig. S2c–d ). The trion quantum yield is then given by: The Auger recombination rate of the biexciton can be expressed as: The PL quantum yield ratio determined from the second-order photon correlation measurement at low fluence is [25] , Using equations (6) and (7), we can extract γ A + knowing QY XX γ r and γ A − . This is how we obtain the values plotted in Supplementary Fig. S2f . Modelling of Auger-assisted photocharging Here we present more details on how we compute the curves in Fig. 3g from the model depicted in Fig. 3h and explained in the main text. We denote the probabilities for the NQD to contain 0, 1 or 2 resident electrons as n 0 , n 1 , n 2 , respectively. The sum of these probabilities is unity: We denote the photo-ionization rate k ion ; it is proportional to the probability of creating a multiexciton: , where P(n,N ex ) is the Poisson probability of exciting an n -exciton when the average number of excitons per NQD is N ex . When the nanocrystal is in a charged state, it relaxes with rates k 1 rel and k 2 rel (singly and doubly charged excitons, respectively; Fig. 3h) . The rate equations for the charging/discharging of the NQD are then written as: We solve these equations for the steady-state regime ( dn i /dt =0; i =0, 1, 2), which describes the time-averaged populations of each charge state and their contributions to PL. Using the notation from the main text and calculating the probability of creating a multiexciton from , we find: where a 1,2 =a ion / k 1,2 rel . These three equations are used to simulate the curves in Fig. 3g . How to cite this article: Galland, C. et al . Lifetime blinking in nonblinking nanocrystal quantum dots. Nat. Commun. 3:908 doi: 10.1038/ncomms1916 (2012).